Polymorphic phase transition mechanism of compressed coesite Silicon dioxide is one of the most abundant natural compounds. Polymorphs of SiO 2 and their phase transitions have long been a focus of great interest and intense theoretical and experimental pursuits. Here, compressing single-crystal coesite SiO 2 under hydrostatic pressures of 26–53 GPa at room temperature, we discover a new polymorphic phase transition mechanism of coesite to post-stishovite, by means of single-crystal synchrotron X-ray diffraction experiment and first-principles computational modelling. The transition features the formation of multiple previously unknown triclinic phases of SiO 2 on the transition pathway as structural intermediates. Coexistence of the low-symmetry phases results in extensive splitting of the original coesite X-ray diffraction peaks that appear as dramatic peak broadening and weakening, resembling an amorphous material. This work sheds light on the long-debated pressure-induced amorphization phenomenon of SiO 2 , but also provides new insights into the densification mechanism of tetrahedrally bonded structures common in nature. As a dominant constituent of the Earth’s crust and mantle and a ubiquitous technological material with an extremely wide range of applications, the structural varieties of silica are of great interest to materials science and geoscience. Coesite, with corner-linked silica tetrahedra (SiO 4 ) in a monoclinic unit cell (space group C 2 /c ), was the first known high-pressure crystalline phase of silica [1] . Its discovery and its transition at higher pressures to stishovite [2] with silicon in octahedral coordination (SiO 6 ) demonstrated the importance of the pressure variable for understanding the deep Earth, and in effect, ushered in the new era of high-pressure mineral physics. Subsequent experiments at higher pressures and high temperatures produced the equilibrium conditions [3] , [4] , [5] , [6] , [7] , [8] , [9] , [10] , and revealed a number of stable post-stishovite phases, including octahedrally coordinated silica with the CaCl 2 and α-PbO 2 structures and eventually to the pyrite structure [11] , [12] , [13] , [14] , [15] , [16] , [17] . The tetrahedron-to-octahedron transition in pure silica also exemplifies the universal phenomena in all silicate minerals throughout the mantle [18] , [19] , [20] . Metastable crystalline and amorphous phases of silica could be equally important and more intriguing than the stable crystalline phases. High pressure and low temperature create conditions that favour the denser packing from 4- to 5- to 6-coordination while hindering the true equilibrium and preserving metastable intermediate states [3] , [21] , [22] . Energy-dispersive X-ray diffraction study of polycrystalline coesite showed the disappearance of sharp crystalline peaks indicating that above 30 GPa silica collapses to an amorphous phase and is metastable up to above 40 GPa at which point an octahedrally ordered phase appears [3] , [6] . However, the possibility of the formation of a fully disordered phase was reputed [23] for lack of long-range atomic diffusion, advocating that a portion of crystal ordering may still be present in the amorphous phase. Furthermore, Car-Parrinello molecular dynamics (MD) simulations [8] predicted a direct phase transition of coesite to an octahedral structure, by pushing the system along the softest mode in the lattice avoiding a collapse of crystalline symmetry. Put comprehensively, the nature of the formation of the intermediate phase is still mysterious and plentiful details remain to be uncovered. Herein lies our motivation for optimizing the experimental protocol and mapping the energy landscape with advanced simulation techniques to unveil the phase transition mechanism of coesite. Experimental results To achieve better sensitivity of the structural determination of silica under high pressure, we adopt the high-pressure single-crystal X-ray diffraction method, and preserve the single crystal and its orientation by using helium as the best hydrostatic pressure transmitting medium. The diffraction patterns from a starting coesite single crystal up to 53 GPa are shown in Fig. 1a–c . At low pressures, all diffraction spots collected on the area detector can be readily indexed with the monoclinic coesite structure ( Fig. 1a ). The sharp coesite diffraction pattern persists up to 26 GPa, when all original coesite diffraction spots split into multiple sharp spots ( Fig. 1b,d ). The spots do not split along constant 2 θ diffraction circles, but across circles with distinct 2 θ values, indicating multiple structures rather than multiple crystals of the same structure. The diffraction pattern after splitting can be uniquely fit into four distinct but nearly isochoric structures ( Fig. 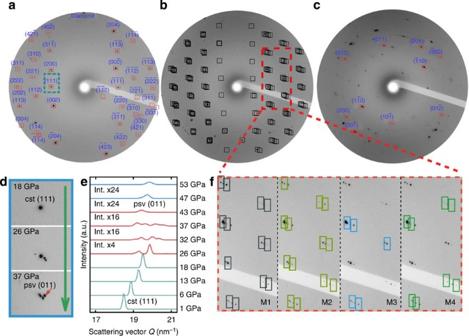Figure 1: X-ray diffraction patterns showing the transition of single-crystal coesite under high pressures. Compressed at (a) 6 GPa, coesite single crystal; (b) 26 GPa, split diffraction patterns of compressed coesite; (c) 53 GPa, crystallized monoclinic post-stishovite (indexed for one grain). (d) Zoomed-in picture corresponding to the (111) diffraction spot ina. The original coesite (111) peak splits into four spots. (e) The evolution of integrated one-dimensional diffraction spectra within the dashed box ina. (f) Four copies of the highlighted diffraction pattern at 26 GPa (b), with the contributions from the four individual metastable structures (M1–M4) highlighted. The abbreviations in the figure: cst, coesite; psv, post-stishovite. 1f ) that each one has a unique orientation matrix and has a topotaxial relationship with the parent coesite crystal ( Supplementary Table 1 ). We note that this phenomenon is in contrast to the reported formation of the intermediate amorphous phase [3] . 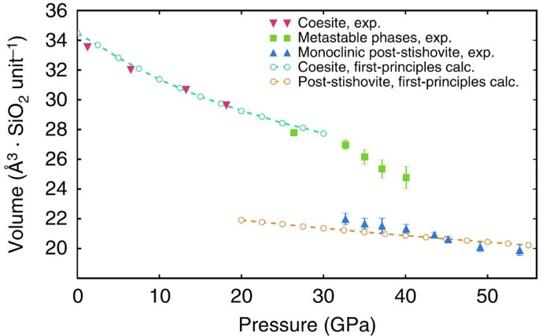Figure 2: The specific volume of coesite as a function of pressure during the compression experiment. The colour markers are: coesite (magenta down triangles), metastable transition intermediates (green squares) and monoclinic post-stishovite (blue triangles). The experimental data are compared with first-principles calculations of the equations-of-state (EOS) of coesite (consistent with the experimental EOS in ref.24) and monoclinic post-stishovite. The error bars indicate the uncertainty in determining the specific volumes of the metastable phases. These phases assume a reduced triclinic symmetry (the structural parameters are shown in Supplementary Table 2 ). The transition results in a large volume collapse (for example, ~4% at 26 GPa) in comparison to the extended equation of states of coesite at this pressure ( Fig. 2 ). Figure 1: X-ray diffraction patterns showing the transition of single-crystal coesite under high pressures. Compressed at ( a ) 6 GPa, coesite single crystal; ( b ) 26 GPa, split diffraction patterns of compressed coesite; ( c ) 53 GPa, crystallized monoclinic post-stishovite (indexed for one grain). ( d ) Zoomed-in picture corresponding to the (111) diffraction spot in a . The original coesite (111) peak splits into four spots. ( e ) The evolution of integrated one-dimensional diffraction spectra within the dashed box in a . ( f ) Four copies of the highlighted diffraction pattern at 26 GPa ( b ), with the contributions from the four individual metastable structures (M1–M4) highlighted. The abbreviations in the figure: cst, coesite; psv, post-stishovite. Full size image Figure 2: The specific volume of coesite as a function of pressure during the compression experiment. The colour markers are: coesite (magenta down triangles), metastable transition intermediates (green squares) and monoclinic post-stishovite (blue triangles). The experimental data are compared with first-principles calculations of the equations-of-state (EOS) of coesite (consistent with the experimental EOS in ref. 24 ) and monoclinic post-stishovite. The error bars indicate the uncertainty in determining the specific volumes of the metastable phases. Full size image With further compression, the diffraction peaks broaden and decrease significantly in intensity. With the split peaks at different 2 θ (or Q ) values, the integrated 1D diffraction spectra become very broad and weak and resemble the amorphization phenomenon reported in the literature [3] . A new set of diffraction peaks from a denser silica phase emerge at 32 GPa and coexist with the existing metastable phases. At these pressures, the resolution of the single crystal diffraction pattern is insufficient to resolve any new distorted crystal structures, which, however, can be mitigated by integrating the spotty patterns into a diffraction spectrum (see Supplementary Fig. 1 ). 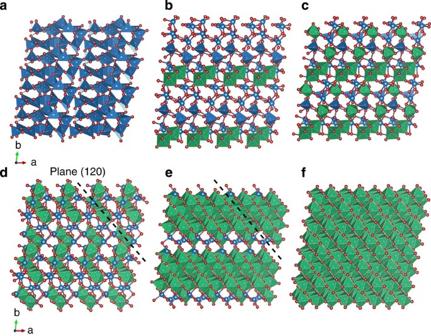Figure 3: Illustration of structural transition from coesite to monoclinic post-stishovite derived fromab initiometadynamics simulation. Structural evolution from (a) coesite to (f) monoclinic post-stishovite phase. (b–e) correspond to the metastable phases (M1–M4) identified from metadynamics simulation, manifesting the SiO6octahedron units (coloured in green) formed along the (120) plane (the SiO4tetrahedron units are coloured in blue). At 40 GPa, the integrated spectra fit a monoclinic post-stishovite structure (space group P 2/ c , for example, Supplementary Table 3 ), corresponding to a density of 4.68 g cm −3 . The new post-stishovite phase was stable up to 53 GPa (the highest pressure achieved in this work) at room temperature and is clearly different from either the monoclinic coesite structure or the triclinic metastable structures at lower pressures. Computational results To elucidate the role of high pressure on the structural changes of coesite, we conducted first-principles MD simulation. The coesite unit cell was gradually pressurized to 40 GPa under a canonical NPT ensemble (constant number of particles, pressure and temperature). The monoclinic structure was slightly distorted but all Si atoms still remain tetrahedrally coordinated by oxygen, corroborating the previously reported compression mechanism of coesite at low pressures [24] . At 40 GPa, the distorted triclinic coesite structure survived long-time ab initio MD simulation (up to 4.8 ps), indicating that an energy barrier prevents further structural changes of coesite and ab initio MD of coesite at 300 K is inadequate to overcome the energy barrier. To circumvent this issue, we employed the metadynamics method [25] , [26] to accelerate sampling of the potential energy surface and probe possible transition pathways of coesite. To this end, the cell edges along the b -axis and the c -axis, together with the sum average of silicon coordination number were used as the collective variables (that is, reaction coordinates) to facilitate barrier crossing. Following the prescribed simulation protocol, within a few hundreds of metasteps, the system undergoes a direct transition from coesite to a monoclinic post-stishovite structure, and four distinct metastable structures are captured along the transition path, exactly matching our experimental observations. The evolution of structure and free-energy landscape is shown in Figs 3 and 4 , respectively. Details about the energetics, lattice parameters and coordination changes during the metadynamics simulation can be found in Supplementary Figs 2 and 3 . Figure 3: Illustration of structural transition from coesite to monoclinic post-stishovite derived from ab initio metadynamics simulation. Structural evolution from ( a ) coesite to ( f ) monoclinic post-stishovite phase. ( b – e ) correspond to the metastable phases (M1–M4) identified from metadynamics simulation, manifesting the SiO 6 octahedron units (coloured in green) formed along the (120) plane (the SiO 4 tetrahedron units are coloured in blue). 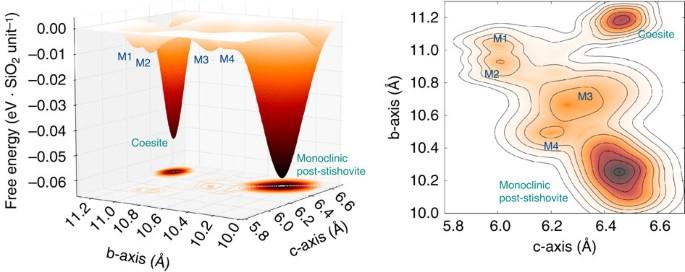Figure 4: Free-energy landscape showing the transition pathway from coesite to post-stishovite. The energy landscape was obtained fromab initiometadynamics simulation at 40 GPa and 300 K (see text) and projected along theb- andc-axis of the unit-cell of SiO2. A hypothetical transition pathway is shown in the right panel (dotted line). Several local energy minima (M1–M4) are present between the stable coesite and post-stishovite phases. The metastability of the various structural intermediates has been confirmed with phonon calculations, where no imaginary vibration modes are identified. Full size image Figure 4: Free-energy landscape showing the transition pathway from coesite to post-stishovite. The energy landscape was obtained from ab initio metadynamics simulation at 40 GPa and 300 K (see text) and projected along the b - and c -axis of the unit-cell of SiO 2 . A hypothetical transition pathway is shown in the right panel (dotted line). Several local energy minima (M1–M4) are present between the stable coesite and post-stishovite phases. The metastability of the various structural intermediates has been confirmed with phonon calculations, where no imaginary vibration modes are identified. Full size image The initial silicon tetrahedral structure distorts and connections between neighbouring silicon atoms are broken after the first 81 metasteps. The system then becomes trapped between two competing metastable structures (for example, see Fig. 4 ), signified by the development of two six-coordinated silicon polyhedra connected perpendicularly to the (110) plane, as shown in Fig. 3b,c . The appearance of the two metastable structures is associated with the unit cell to shorten by 7.7% along the c -axis. The new structural motifs with five- and six-coordinated polyhedra stabilize the lattice. With prolonged metadynamics simulation, more six-coordinated silicon atoms form along the (120) plane, resulting in an expansion of the c -axis and compression of the b -axis. Correspondingly, two more metastable structures with similar enthalpies are identified from the small dips M3 and M4 in Fig. 4 , where silicon octahedra are aligned alternately along the (120) plane. The coordination change along the metadynamics simulation, illustrating the reconstructive nature of the phase transition, is shown in Fig. 3 . The newly discovered transition mechanism of compressed coesite is different from what was reported by Martonák et al . [8] , [9] . It is interesting to note that all the four metastable phases emerging from ab initio metadynamics (M1–M4) contain fivefold coordinated Si atoms. The fivefold silicon coordination has been speculated before, but has never been experimentally confirmed. We thus set out to verify the stability of the metastable structures populated with fivefold Si coordination through ab initio MD simulation. The metastable structures are further quenched to 26 GPa and 0 K for phonon dispersion calculations (see Supplementary Fig. 4 ). No imagery vibration modes are found for those transition intermediates in the Brillouin zone, confirming they are indeed metastable in the pressure range of interest. These metastable phases match the experiment results in the same pressure range (26–40 GPa), in which the four sets of diffraction patterns can be explained by the formation of the metastable structures in an on-going phase transition. Two of the metastable structures from our experiment also show that the lattice parameter in the b -axis continues to decrease and the c -axis is greatly softened, which is exactly reproduced by our simulation. In our ab initio metadynamics simulation, the lattice parameters of the resulting monoclinic post-stishovite are comparable with the experimental data ( Supplementary Table 3 ). At no point was a disordered or amorphous phase observed through these simulations, in line with our experimental observations. The re-coordination of silicon atoms, driven by the instability of SiO 4 tetrahedron short-range ordering structures at high pressure (>26 GPa) has a preferred formation plane along (120) in the coesite unit cell. The phase transition from tetrahedrally coordinated low-pressure silica phases to octahedrally coordinated phase is a thermally activated process. Owing to the energy barriers separating the different energy wells on the energy landscape, the metastable phases coexist and render the transition from coesite to post-stishovite a slow kinetic process, which explains the broad span of pressures (from 26 to 40 GPa) over which the transition is found to occur in the experiment. In summary, using the integration of hydrostatic single-crystal X-ray diffraction, multiple crystal analytical technique and ab initio computer simulation, we made several surprisingly important discoveries, which may help resolve the long-standing enigma of pressure-induced amorphization of coesite. We observed four new triclinic structures of SiO 2 that have not been reported or calculated previously, and found the long sought for five-coordinated Si in all four new phases. We conclude that the ostensible amorphous mixture may result from the coexistence of the low-symmetry crystalline phases en route from Si tetrahedra to octahedra. The multiple metastable phases on the transition pathway constitute the true phase transition mechanism from four-cordinated to six-coordinated silica. Last, our results demonstrate the power of this integrated low-temperature approach to freeze in intermediate phases and garner true understanding of the transition mechanism of refractory materials. High-pressure single-crystal X-ray diffraction experiment Multiple X-ray diffraction experiments were performed on coesite single crystals. Experiments were performed at beamline number 16 ID-B/BM-D of High-Pressure Collaborative Access Team (HPCAT) of the Advanced Phonon Source, Argonne National Laboratory. Thin-cut synthetic coesite single-crystal samples (~30 μm ( L ) × 30 μm ( W ) × 10 μm ( T )) [27] were loaded in Mao-Bell diamond anvil cells [28] . The samples were loaded into tungsten gaskets with helium gas as the pressure medium. Diffraction patterns were collected at each X-ray incident angle from −15° to 15° (1° per image) and another image was taken continuously for the same scanned range. The orientation matrix and crystalline structure were calculated by the difference vector approach. Pressure was determined by calibrating the ruby fluorescence line shift in an offline Ruby system. The uncertainty in the pressure was ±0.8 to 1.9 GPa, derived from the pressure change within each experiment interval. For all experiments, we have conducted on coesite, consistent diffraction patterns were reproduced at all pressures and room temperature using multiple samples. Compression rate in the high-pressure X-ray diffraction experiment The compression rate may have an effect on the high-pressure phase behaviour of single-crystal samples due to kinetic considerations. In our experiments, the pressurization process is considered as quasi-static. The pressure was applied by manually tightening the screws of the DAC off the beamline. A typical pressure increment during the transition regime is 2–3 GPa per run, monitored by the line-shift in an off-line ruby system that calibrates the pressure. This was achieved by symmetrically and slowly tightening the screws and the pressure was slowly increased to equilibrium within 5–10 min (corresponding roughly to 0.5 GPa min −1 in terms of compression rate). The diffraction patterns were taken after the pressure was stabilized. A typical cycle for collecting each diffraction pattern is around 45 min. The pressure was re-measured after each diffraction experiment, and the changes of the pressure were used as the uncertainties of pressure measurements. The structures obtained at high pressures may be susceptible to high compression rates, which, however, has yet to be thoroughly investigated. Using helium gas as the pressure medium Helium gas was used as the pressure medium in our experiments. It has been pointed out previously that the injection of helium atoms into large interstitial sites make occur in SiO 2 glass [29] , [30] , cristobalite [31] and zeolite [32] . For example, in SiO 2 glass and cristobalite, helium atoms can penetrate into the six-membered rings. However, coesite forms four-membered rings, which have relatively smaller interstitial spatial sites (ISSs). At ambient conditions, the coesite ISSs are 53% smaller than cristobalite’s measured in volume, which renders it rather difficult for helium atoms to penetrate into the ISSs of coesite. Experimentally, the penetration of He atoms into the solids would result in noticeable changes of the compressibility of the materials [29] , [30] . In our experiment, all diffraction peaks shifts normally, and no dramatically changes of compressibility of coesite were found. The experimental equations-of-state of coesite also matches our first-principles simulation, which is independent on pressure medium. We therefore conclude that the compression behaviour of coesite is not affected by the pressure medium used in this work. First-principles computer simulation Ab initio MD simulations were performed using the Car-Parrinello Molecular Dynamics (CPMD) package [33] . A single-unit cell of coesite (16 silicon atoms+32 oxygen atoms with periodic boundary conditions) was used in the MD simulation following the ab initio Car-Parrinello scheme, together with a perturbative potential as prescribed by the metadynamics method [25] , [26] . We employed the combination of the Becke exchange functional [34] and the Lee-Yang-Parr correlation functional [35] as the exchange-correlation energy, parameterized by Goedecker et al . [36] A typical kinetic cutoff of 150 Ry was used in MD simulations. We used 2 a.u. (0.05 fs) for each MD timestep. The metadynamics simulations were carried out under a constant pressure and constant temperature (NPT) ensemble. A Gaussian type bias energy, with its shape optimized for different phase regions was added at each metastep, followed by an equilibration run using ab initio MD. Equations-of-state and phonon calculations were performed with the Quantum Espresso code [37] adopting the above-mentioned pseudopotentials and the same energy cutoff. Description of ab initio metadynamics simulation Metadynamics simulations were performed with the CPMD package [33] . A coesite unitcell (48 atoms, space group C 2/ c ) was initially compressed to 40 GPa, and equilibrated for 2 ps at 300 K with ab initio MD in an NPT ensemble [38] with the Parrinello-Rahman Lagrangian algorithm [39] . During ab initio MD simulation, the fluctuations of fictitious electron kinetic energy were restricted by a velocities scaling in a range of ±300 K, whereas the nuclear degree of freedom was controlled by the Nosé-Hoover chain thermostats [40] . For metadynamics simulation, various combinations of collective variables (CVs) have been carefully tested. In this work, the most effective CVs were chosen to be the cell-edges (lengths) of b and c axes as well as the average coordination number of silicon atoms. The coordination number is defined as: where d ij refers to Si–O bond distance; d 0 is a reference bond length (2.1 Å); i and j loop over silicon and oxygen atoms, respectively. Consequently, the bias energy V ( s , t ) along the metadynamics simulation is given by: where t denotes simulation time and s i is the value of the i th CV. The height ( h ) and width of the Gaussian hill shape were discretely selected to facilitate our metadynamics simulation. The fluctuations of all CVs were first monitored without modifying the free-energy landscape. These try runs enabled us to determine the energy scaling factors to synchronize all CVs , satisfying the equation: where ω i is the fluctuation range for the i th CV. The Gaussian width δ s was set to be ¼ of the fluctuation of a CV type and applied to all CVs by multiplying their scaling factors. The height of the Gaussian type bias energy was chosen within 0.5–2.0 k B T, depending on the phase regions the simulation samples (A shallower height, for example, 0.5 k B T, was applied near the saddle point of the phase transition). Such potential heights were proven efficient in filling most energy wells in similar simulations [41] , [42] . After a bias energy was deposited at each metastep, the system was equilibrated with lengthy ab initio MD simulation. The number of MD steps was determined in such a way that the CV displacement is comparable with the width of the bias energy, avoiding the so-called ‘hill surfing problems’ [43] . Therefore, the metadynamics timestep was chosen adaptively such that a Gaussian is placed at t i once the following condition is fulfilled: As soon as a phase transition was identified, the energy deposition parameters were updated. The parameters used in sampling SiO 2 polymorphs at 40 GPa and 300 K are briefly summarized in Supplementary Table 4 . In Fig. 4 , the derived free energy landscape was projected along cell edge b ( s 1 ) and c ( s 2 ). At each metastep, a two-dimensional Gaussian-type energy was added to the energy landscape. The energy intensity z as a function of s 1 and s 2 is calculated by: How to cite this article: Hu, Q. Y. et al . Polymorphic phase transition mechanism of compressed coesite. Nat. Commun. 6:6630 doi: 10.1038/ncomms7630 (2015).